Visualization of nanocrystal breathing modes at extreme strains Nanoscale dimensions in materials lead to unique electronic and structural properties with applications ranging from site-specific drug delivery to anodes for lithium-ion batteries. These functional properties often involve large-amplitude strains and structural modifications, and thus require an understanding of the dynamics of these processes. Here we use femtosecond X-ray scattering techniques to visualize, in real time and with atomic-scale resolution, light-induced anisotropic strains in nanocrystal spheres and rods. Strains at the percent level are observed in CdS and CdSe samples, associated with a rapid expansion followed by contraction along the nanosphere or nanorod radial direction driven by a transient carrier-induced stress. These morphological changes occur simultaneously with the first steps in the melting transition on hundreds of femtosecond timescales. This work represents the first direct real-time probe of the dynamics of these large-amplitude strains and shape changes in few-nanometre-scale particles. Although extensive investigations have been carried out probing modifications in the electronic, thermodynamic and kinetic properties of semiconductor quantum dots as a function of size and shape, the size-dependent structural dynamics exhibited by nanocrystals are not well understood. For example, surface energies play a crucial role in nanoparticle phase stability, leading to size-dependent modifications of solid–liquid [1] , [2] or solid–solid [3] , [4] transition temperatures, but the dynamics of these transformations have not been resolved using techniques providing both atomic-scale and femtosecond resolution, the relevant length and timescales for these processes. The elastic properties and stress and strain response exhibited by nanocrystals are size dependent with novel mechanical properties emerging at the nanoscale, associated with variations in bulk moduli and the ability to withstand extreme stresses without inelastic or plastic responses [5] , [6] , [7] , [8] , [9] . These properties have been utilized in the development of nanowire electrochemical cells in which ion-induced transformations are markedly modified compared with the bulk [10] and in the engineering of nanoscale thin films or two-dimensional materials with unique strain-induced structural phases [11] , [12] . In turn, these mechanical properties and associated anisotropic response or shape changes are intrinsically linked to the functionality and stability of nanoscale optoelectronic and nanoelectromechanical devices. As such, a real-time probe sensitive to atomic length-scale rearrangements and nanoscale morphological changes is required to elucidate their dynamical and functional response in-situ [13] , [14] , [15] . Time-resolved approaches utilizing optical probes have been applied previously to elucidate the elastic and acoustic response exhibited by nanomaterials. Optical pump-probe studies indirectly reflect structural responses and show evidence for breathing and extensional mode excitations, with typical periods of order 1 ps associated with sound–velocity-limited strains at the nanoscale (1 nm/(1,000 m s −1 )~1 ps; refs 16 , 17 , 18 , 19 ). X-rays have been used to map the acoustic response of few hundred nanometre particles on hundreds of picosecond timescales [20] , [21] , [22] . Here we use femtosecond X-ray scattering techniques to visualize the anisotropic shape changes and deformations in the limit of large strains and on femtosecond timescales. Measurement of multiple nanocrystal diffraction peaks enables the photoinduced time-dependent strains to be projected along the relevant axes of the nanostructure, independent of its orientation. For both nano-sized spheres and rods, we show that intense above-bandgap photoexcitation leads to percent level radial expansions occurring on few hundred femtosecond timescales. These are followed by a reversible contraction, with the nanocrystals exhibiting a quasi-half-cycle acoustic response. For the case of an anisotropic nanorod, we show that the expansion is anisotropic as well, with the expansion occurring only along the radial direction of the nanorod at short times, as reflected directly in the variation in the time-dependent amplitudes for different diffraction peaks. Quantitative modelling of the observed strain response for both spheres and nanorods shows that the first steps in the structural response are driven by electronic stresses rather than thermal ones, under conditions of order 1,000 electron–hole pairs/nanocrystal. Simultaneously, in this work, we resolve the structural dynamics associated with the first steps in the semiconductor nanocrystal melting process, which occur concurrently with the ultrafast strain response. 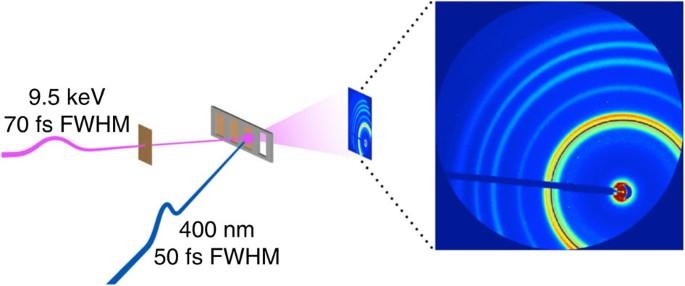Figure 1: Schematic of the experimental setup. Femtosecond X-ray pulse passes through X-ray timing monitor and then diffracts from ~100-nm-thick nanocrystal powder on a Si3N4membrane in a transmission geometry following above-bandgap femtosecond laser excitation. Snapshots of the time-resolved diffraction pattern are recorded on a large-area detector read out on a shot-by-shot basis. At right is raw diffraction image from CdS nanorods. FWHM, full-width at half-maximum. Experimental setup Figure 1 shows a schematic of the experimental setup: 70 fs full-width at half-maximum 9.5 keV ( λ =1.3 Å) X-ray pulses generated at the Linac Coherent Light Source [23] pass through a timing monitor to record the relative arrival time between pump and probe [24] , before diffracting from a photoexcited 100-nm-thick layer of nanocrystals deposited with random orientation on a thin SiN membrane in transmission geometry (see Methods section). Also shown in Fig. 1 are raw diffraction patterns from CdS nanorods as recorded on an area detector. 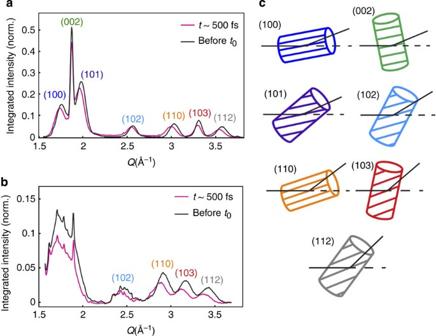Figure 2: Nanocrystal X-ray scattering data. (a) Azimuthally integratedQ-dependent scattering pattern from 18 × 4.5 nm CdS nanorods shown att=0 (black) andt=500 fs (magenta). Miller indices are indicated for all reflections. (b) As above for CdSe 3.4 nm diameter spheres. Narrow peaks associated with organic surfactants are superimposed on the merged-together lowQreflections. (c) The orientation of each set of lattice planes probed shown with respect to the nanorodcaxis, and the orientation of the nanocrystal with respect to the incident and outgoing X-ray wave vectors. Norm., normaliz`ed. Figure 2 shows sample X-ray diffraction patterns for both 3.4 nm diameter CdSe spheres and 4.5 × 18 nm CdS rods recorded before and 500 fs after excitation by above-bandgap 400 nm wavelength optical pulses with a laser fluence of 0.4 J cm −2 ( Supplementary Note 1 ). The first seven allowed peaks of the hexagonal wurtzite structure are collected for both morphologies, with the sharp (002) reflection for the rod samples indicating that the long axis of the nanorod corresponds to the c axis of the hexagonal unit cell [25] . The orientations for all measured lattice planes/reflections are shown as well in Fig. 2 . For both the spherical and rod samples, changes in the diffraction intensity, associated with disordering processes, are superimposed on homogeneous shifts of the diffraction peaks to lower Q (=4 π sin θ / λ , where 2 θ is the scattering angle shown in Fig. 2c . Figure 1: Schematic of the experimental setup. Femtosecond X-ray pulse passes through X-ray timing monitor and then diffracts from ~100-nm-thick nanocrystal powder on a Si 3 N 4 membrane in a transmission geometry following above-bandgap femtosecond laser excitation. Snapshots of the time-resolved diffraction pattern are recorded on a large-area detector read out on a shot-by-shot basis. At right is raw diffraction image from CdS nanorods. FWHM, full-width at half-maximum. Full size image Figure 2: Nanocrystal X-ray scattering data. ( a ) Azimuthally integrated Q -dependent scattering pattern from 18 × 4.5 nm CdS nanorods shown at t =0 (black) and t =500 fs (magenta). Miller indices are indicated for all reflections. ( b ) As above for CdSe 3.4 nm diameter spheres. Narrow peaks associated with organic surfactants are superimposed on the merged-together low Q reflections. ( c ) The orientation of each set of lattice planes probed shown with respect to the nanorod c axis, and the orientation of the nanocrystal with respect to the incident and outgoing X-ray wave vectors. Norm., normaliz`ed. Full size image Sphere and rod response Focusing first on the case of the nanosphere response, Fig. 3 shows the time dependence of the normalized angular peak shifts Δ Q / Q ( t ) for all measured reflections in a few picosecond time window. All reflections are observed to have the same normalized shift within experimental error. This independence on the crystallographic direction within the sphere implies a radially symmetric strain as would be expected for an acoustic radial breathing mode. The magnitude of the peak shift indicates a maximum photoinduced strain of ~1.2% (Δ d / d =−Δ Q / Q where d is a lattice spacing) corresponding to strain rates of ~2 × 10 10 s −1 . The period of the acoustic breathing mode excitation in a spherical nanocrystal is T =2 πR /( χc L ) in a continuum approximation, where R is the nanocrystal radius, χ is the first solution of the equation tan χ = χ /(1− c L 2 χ 2 /4 c T 2 ), and c L and c T are the longitudinal and transverse wave velocities, respectively [26] . Using known values for bulk CdSe [27] , this gives a period of ~1.1 ps in qualitative agreement with the observed response. This simple model does not account for the effects of the surrounding matrix but is in reasonable agreement with prior measurements [17] . The inset to Fig. 3a shows the long-time response ( t =60 ps) showing no long-lived strain induced within the signal to noise of the measurement. The observed effects for the nanospheres are therefore indicative of an isotropic radial breathing mode associated with an expansion and then contraction to the initial diameter, corresponding to one-half of an acoustic cycle. 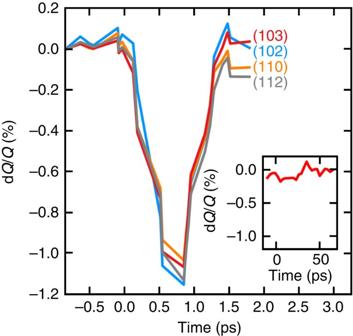Figure 3: Sphere radial breathing response. dQ/Qfor 3.4 nm CdSe spheres for reflections indicated, showing isotropic breathing mode response with dynamics independent of the reflection probed (inset): long-time response showing no long-lived-induced strain. Figure 3: Sphere radial breathing response. d Q / Q for 3.4 nm CdSe spheres for reflections indicated, showing isotropic breathing mode response with dynamics independent of the reflection probed (inset): long-time response showing no long-lived-induced strain. Full size image In contrast to the case of the spheres where Δ Q / Q is independent of the particular X-ray reflection, the nanorod response shows a complex dependence on (hkl) ( Fig. 4a ), with smallest effects observed for the (002) reflection, corresponding to planes orthogonal to the long axis and no obvious dependence on Q hkl . This is indicative of an anisotropic response in which changes in the interlayer lattice spacing are dependent on their orientation with respect to the nanocrystal axes. By recording peak shifts for each reflection, we are able to reconstruct the anisotropic shape changes within the nanorod by effectively projecting the time-dependent strains along different axes of the nanostructure. We show in the following that the observed short-time response is fully consistent with a pure radial expansion of the nanowire, as observed for the case of the spheres above. 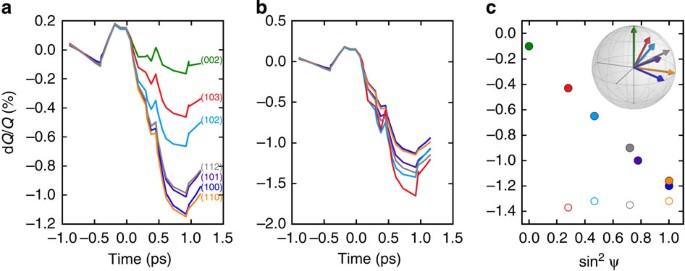Figure 4: Nanorod anisotropic response. (a) Nanorod time-dependent shift dQ/Qfor reflections indicated showing anisotropic response. (b) Data inascaled by factor sin2ψhklwhere ψhklis the angle between the lattice planes with indices (hkl) and the long axis of the nanorod. (c) dQ/Qfor sphere (open circles) and rod (closed circles) samples as a function of sin2ψhkl. Colours match the labelled colours at left. Inset shows different tomographic views with the long axis of the nanorod (in green) along thecaxis. Figure 4: Nanorod anisotropic response. ( a ) Nanorod time-dependent shift d Q / Q for reflections indicated showing anisotropic response. ( b ) Data in a scaled by factor sin 2 ψ hkl where ψ hkl is the angle between the lattice planes with indices (hkl) and the long axis of the nanorod. ( c ) d Q / Q for sphere (open circles) and rod (closed circles) samples as a function of sin 2 ψ hkl . Colours match the labelled colours at left. Inset shows different tomographic views with the long axis of the nanorod (in green) along the c axis. Full size image During a radial expansion, different sets of lattice planes experience different acoustic strains. For example, the (002) planes, lying perpendicular to the long axis of the nanorod, have no component along the radial direction and will experience no change in d-spacing. In contrast, the (100) and (110) planes, which are perpendicular to the radial direction, sense the radial breathing mode fully, as observed. In order to understand the response of the other reflections, consider the strain experienced by lattice planes with arbitrary angle ψ hkl with respect to the (002) planes ( Supplementary Fig. 1 ). This effect has been considered before with respect to scattering from asymmetric reflections in solids under strains normal to the surface and for uniaxial shocks and can be accounted for by including a factor of sin 2 ψ hkl in the relation between the strain and the fractional change in Q [15] , [28] , [29] ( Supplementary Note 2 and Supplementary Table 1 ). Thus, the influence of a radial strain on the lattice spacing associated with reflection (hkl) can be written: where ε is the radial strain, d hkl is the lattice spacing for reflection (hkl), c is the hexagonal c axis lattice constant and the right-most result is specific for the case of a hexagonal unit cell. This has the correct dependence as seen by the limiting cases for ψ 002 =0 and ψ 100 = ψ 110 = π /2. More generally, scaling the data after time zero for each (hkl) by the factor sin 2 ψ hkl collapses the complex response shown in Fig. 4a onto a single curve directly showing the time-resolved nanowire radial strain ( Fig. 4b ). Alternatively, plotting the peak magnitude (at t ~800 fs) of Δ Q / Q hkl as a function of sin 2 ψ hkl shows the expected linear dependence with slope equal to the magnitude of the radial strain, ~1.2% ( Fig. 4b ), consistent with a radial expansion as observed for the spherical geometry as shown in Fig. 4c . Together, these results show that the dynamical response of the nanowire is anisotropic, with the dominant strain associated with a radial expansion of the nanowire with no long-lived strain observed ( Supplementary Fig. 2 ), as in the case of the spheres. Some small variation in the curves shown in Fig. 4b indicates that this model does not capture all aspects of the dynamical shape changes, but it clearly does capture the most relevant aspects. The observed timescales for this expansion are in agreement with expected values (see Methods section). At short times, this anisotropic response is as expected: extensional modes will turn on on timescales of order 10 ps but these compete with the simultaneous disordering processes discussed below. We observe that concurrently with the strain responses discussed above, the photoexcitation conditions used in this experiment are sufficient to drive ultrafast disordering processes within the nanocrystals, as reflected in changes in the peak intensity or integrated area of the diffraction peaks. These additional structural responses provide a means, moreover, to understand the surprising strongly damped acoustic response shown above. 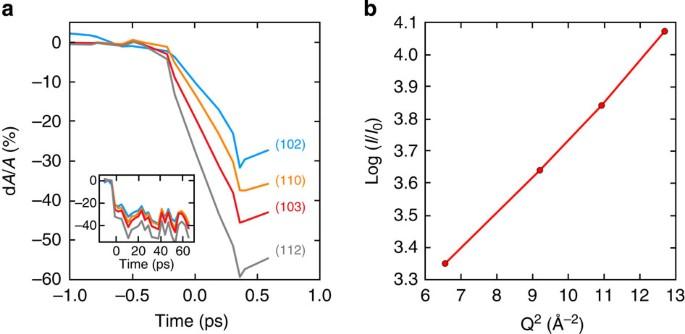Figure 5: Sphere disordering/melting dynamics. (a) Short timescale change in integrated area for the indicated reflections. (Inset) Long-time response showing long-lived reductions in diffracted intensity. (b) Debye–Waller fit showing logarithm of normalized scattered intensity versusQ2att=400 fs. Figure 5 shows time scans of the normalized integrated area d A / A for the four highest Q reflections of the 3.4-nm spheres. The timescales for the disordering process are comparable to the observed strain-induced expansion dynamics and consistent with similarly fast disordering timescales observed in bulk semiconductors [30] , [31] , [32] , [33] not previously measured for the case of semiconductor nanocrystals. In contrast with the breathing mode response, the changes in integrated area persist out to the longest times probed (8 ns) ( Fig. 5 inset and Supplementary Figs 3 and 4 ). In addition, the Q dependence of the disordering/melting response is significantly simpler than for the strain/breathing response, showing larger amplitude effects for larger Q for both spheres and rods as would be expected according to a Debye–Waller-like model, for example, I ( Q , t )= I o exp(− Q 2 σ ( t ) 2 /3), where σ ( t ) is the time-dependent root mean square displacement (r.m.s.d.) of the atoms [30] . A plot of the dependence of log( I ( t )) on Q 2 at t =400 fs ( Fig. 5b ) demonstrates the data’s consistency with this model showing a linear dependence. We extract from the slope of this plot an r.m.s.d. of ~0.6 Å, comparable to the maximum radial strain-induced change in the sphere diameter and a large fraction of an interatomic spacing [34] . Similar behaviour is observed for the rod samples ( Supplementary Figs 3 and 4 ). Given this information, the half-cycle acoustic response observed for the nanosphere radial breathing mode can likely be attributed to ultrafast phonon-scattering processes. These scattering processes impact the population and coherence of the induced elastic standing wave within each nanocrystal, with the scattering rates strongly increasing as a result of the extreme disorder both at the surface and within the nanocrystal. Estimates based on prior theoretical models [35] suggest that at temperatures of ~1,000 K (comparable to those induced within each nanocrystal— Supplementary Note 1 , and Supplementary Figs 5 and 6 ), these scattering rates are of order 1 THz (with scattering mean free paths comparable to the nanocrystal diameter), which is consistent with the strongly damped coherent response observed. Similar acoustic damping effects in strongly photoexcited semiconductor thin films have been observed by X-ray techniques [36] and by optical pump-probe techniques [17] . The observed damping is inconsistent with dephasing associated with the finite size distribution of the nanocrystals ( Supplementary Note 3 ). Because long-lived strain responses are not observed within the signal to noise of the measurement (for both spheres and rods; Fig. 3 inset and Supplementary Fig. 2 ), the applied stress must be transient, which implies a direct carrier-induced rather than temperature-driven trigger for both the disordering process and the initial breathing mode response [37] , [38] . This is consistent with previous studies in bulk semiconductors that indicate a large-amplitude carrier-induced stress at short times under femtosecond excitation conditions, with the electronic stress dominating over the thermal stress [39] . For temperature jumps of ~1,000 K, the peak strain using bulk values for the thermal expansion coefficient [27] is ~3 × smaller than the peak strain measured here and likely not resolvable within the signal to noise of the measurement ( Supplementary Note 1 ). Figure 5: Sphere disordering/melting dynamics. ( a ) Short timescale change in integrated area for the indicated reflections. (Inset) Long-time response showing long-lived reductions in diffracted intensity. ( b ) Debye–Waller fit showing logarithm of normalized scattered intensity versus Q 2 at t =400 fs. Full size image Using this model, one may quantitatively fit the observed acoustic response shown in Fig. 3 to a forced simple harmonic oscillator model with damping, following previously proposed models for coherent excitation of acoustic modes in nanocrystals [18] , [40] . Here the nanocrystal displacement follows the equation: with x a measure of the radial strains/displacements, σ proportional to a time-dependent stress turning on at time zero and τ D an effective damping time. 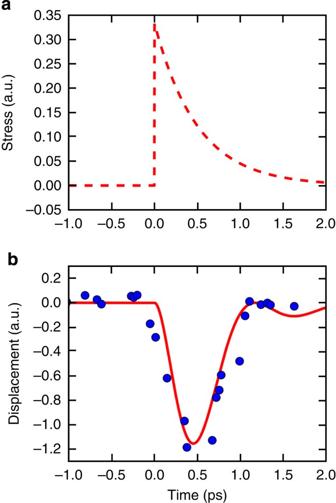Figure 6: Nanocrystal time-dependent stress. (a) Estimated time-dependent stress associated with acoustic breathing mode. (b) Calculated radial displacements (solid line) compared with measured data (points). Figure 6 shows best fit for the time-dependent stress and the corresponding time-dependent displacement calculated from this equation shown in comparison with the measured data for the 3.4-nm CdSe acoustic response. Good agreement is obtained for decay times and damping times of ~500 fs. Here the damping reflects both scattering from the induced disorder as well as coupling of the nanocrystal to the surrounding matrix. A 500-fs decay time for the applied stress is in agreement with prior studies of the ultrafast relaxation of photoexcited carriers in CdSe nanocrystals of this size: electron–hole–hole Auger processes lead to sub-picosecond timescale coupling to the lattice typically through hole relaxation without phonon bottleneck effects [38] , [41] , [42] . Figure 6: Nanocrystal time-dependent stress. ( a ) Estimated time-dependent stress associated with acoustic breathing mode. ( b ) Calculated radial displacements (solid line) compared with measured data (points). Full size image In conclusion, this work represents the first measurements of the femtosecond structural dynamics exhibited by nanocrystals in the limit of extreme strains, directly resolving the ultrafast anisotropic strain and disordering dynamics, and their coupling. New opportunities for all-optical tuning of the dynamic functionality of nanoscale devices may emerge as a result of this work. The analysis presented additionally allows for the in situ characterization of atomic length-scale dynamics along different crystallite directions in nanostructures with anisotropic morphologies, regardless of their orientation in space. Experimental Experiments were carried out at the Linac Coherent Light Source X-ray pump-probe hutch using hard X-ray scattering in a collinear transmission geometry at the undulator fundamental at 9.5 keV X-ray energy [23] ( Fig. 1 ). X-ray pulses with 70 fs full-width at half-maximum pulse duration were used with the diffraction patterns recorded on a large-area MAR detector. Fifty-femtosecond optical pulses with a central wavelength of 400 nm were used to photoexcite (above bandgap) a thin ~100 nm layer of CdSe or CdS nanocrystals in spherical or rod morphology spin coated onto an array of Si 3 N 4 membranes with random orientation as evidenced by the azimuthal symmetry of the diffraction patterns ( Fig. 1 ). Samples were synthesized according to literature procedures [25] and precharacterization was carried out by transmission electron microscopy (TEM) ( Supplementary Figs 7–9 ). Spectral encoding of the relative delay between the optical pump pulse and free electron laser (FEL) probe pulse enabled ~100 fs resolution of the measured nanocrystal dynamics [24] . Single-shot X-ray diffraction patterns were collected of the nanocrystal dynamical response, and the target array was translated subsequent to each shot in order to study a fresh nanocrystal sample at all times. For each relative time delay, measurements of the static unpumped diffraction pattern were made before laser excitation using 100 X-ray shots at 1% of the peak intensity to account for sample inhomogeneity without damaging the samples before each measurement. For extraction of time-resolved changes in diffracted intensity, additional normalization of the diffraction patterns to variations in the X-ray shot-to-shot intensity was carried out using the low Q scattering from each sample position. The diffractograms were azimuthally integrated and fit to extract integrated intensity and peak position. No significant azimuthal dependence to the observed dynamics was observed. Calibration of the diffraction patterns was carried out using a LaB 6 reference sample placed in the same plane as the nanocrystal samples. For quantitative extraction of peak shifts and changes in peak area, the azimuthally integrated Q -dependent diffraction pattern was fit to the sum of Gaussians with adjustable width and position in Q space. Breathing mode formula for a nanowire Under photoexcitation of a nanorod of radius r , the short timescale strain response is expected to be dominated by radial expansion dynamics because of the longer required time for strains to develop along the long axis of the rod. At low excitation fluences, the expected response, following previous studies, consists of radial breathing modes with frequencies where τ n satisfies the eigenvalue equation and where E is Young's modulus, ρ is the density and ν is Poisson’s ratio [43] , [44] . Using tabulated values [27] , we calculate a period of ~1.6 ps for a 4.5-nm CdS nanowire. Similar values are obtained for the case of the spherical geometry. Diffraction analysis Supplementary Note 2 derives the key relation of this paper, encoding the relationship between the observed angular shift of a nanocrystal reflection (hkl) and the angle ψ between this set of lattice planes and the planes normal to the c axis growth direction. For the case of a hexagonal unit cell, the angle between two sets of planes indexed by Miller indices (h 1 ,k 1 ,l 1 ) and (h 2 ,k 2 ,l 2 ) is given by [45] : This relation is used to calculate the relevant angles between the vectors [hkl] and [002]. Supplementary Table 1 gives the calculated values for all reflections used in this paper. How to cite this article: Szilagyi, E. et al . Visualization of nanocrystal breathing modes at extreme strains. Nat. Commun . 6:6577 doi: 10.1038/ncomms7577 (2015).